Ecscr regulates insulin sensitivity and predisposition to obesity by modulating endothelial cell functions Insulin resistance is closely associated with obesity and is one of the earliest symptoms of type-2 diabetes. Endothelial cells are involved in the pathogenesis of insulin resistance through their role in insulin delivery and adipose tissue angiogenesis. Here we show that Ecscr (endothelial cell surface expressed chemotaxis and apoptosis regulator; also known as ARIA), the transmembrane protein that regulates endothelial cell signalling, is highly expressed in white and brown adipose tissues, and regulates energy metabolism and glucose homeostasis by modulating endothelial cell functions. Ecscr-deficient mice fed a normal chow show improved glucose tolerance and enhanced insulin sensitivity. We demonstrate that Ecscr deletion enhances the insulin-mediated Akt/endothelial nitric oxide synthase activation in endothelial cells, which increases insulin delivery into the skeletal muscle. Ecscr deletion also protects mice on a high-fat diet from obesity and obesity-related metabolic disorders by enhancing adipose tissue angiogenesis. Conversely, targeted activation of Ecscr in endothelial cells impairs glucose tolerance and predisposes mice to diet-induced obesity. Our results suggest that the inactivation of Ecscr enhances insulin sensitivity and may represent a new therapeutic strategy for treating metabolic syndrome. The epidemic of obesity and type-2 diabetes are the major health problems worldwide, both of which increase the risk of developing cardiovascular disease [1] , [2] . The earliest defect in developing type-2 diabetes is the reduced metabolic action of insulin in peripheral tissues, namely insulin resistance [3] . Insulin resistance induces the endothelial cell (EC) dysfunction through hyperglycaemia, hyperinsulinaemia and increased circulating free fatty acid concentrations [4] , [5] , [6] , [7] . Endothelial dysfunction causes the disruption of vascular integrity, resulting in the increased cardiovascular morbidity and mortality. On the other hand, EC is an insulin target as well, and insulin-mediated signals modify various EC functions. Insulin signalling in EC modulates endothelial apoptosis and nitric oxide (NO) production, and it attenuates the progression of atherosclerosis [8] , [9] . Recently, an insulin-mediated Akt/endothelial NO synthase (eNOS) activation was shown to have an essential role in insulin delivery into the interstitium of the skeletal muscle that accounts for ~90% of whole-body glucose disposal in human [10] , [11] . Therefore, insulin signalling in EC is also one of the important factors regulating systemic insulin sensitivity. Obesity is closely associated with insulin resistance by initiating the white adipose tissue (WAT) inflammation that alters the secretion of adipocytokines affecting glucose homeostasis [12] . The healthy WAT expansion accompanies the proper neovessel formation, but excessive adiposity triggers adipose tissue hypoxia due to imbalanced vascularization and results in chronic inflammation in WAT, leading to the obesity-related metabolic disorders [13] . In contrast, the brown adipose tissue (BAT) is a thermogenic organ, and its high degree of specialization of lipolysis and fatty acid oxidation allows it to make a major contribution to the overall energy balance [14] . Oxygen consumption in BAT is enormously high; hence, its thermogenic activity can counteract the obese phenotype [13] . The high thermogenic activity of BAT requires a particularly high rate of blood perfusion, and because of this functional requirement BAT contains an extraordinarily well-developed vascular networks. Moreover, a strong correlation between the blood vessel density in BAT and the capacity of thermogenesis and metabolic rate has been reported [15] , [16] , [17] . Therefore, angiogenesis in WAT and BAT is a crucial factor in the pathogenesis of obesity and its related metabolic disorders. EC has a fundamental role in postnatal angiogenesis as well, and thus EC functions are crucially involved in the regulation of energy metabolism and glucose homeostasis, whereas the detailed mechanisms regulating the endothelial insulin signalling and adipose tissue angiogenesis remain to be elucidated. We and others recently identified a previously uncharacterized gene, termed Ecscr (EC surface expressed chemotaxis and apoptosis regulator; also known as ARIA), which is highly preferentially expressed in ECs and controls neovessel formation by regulating the endothelial PTEN (phosphatase and tensin homologue deleted from chromosome 10)/PI3K (phosphoinositide 3-kinase) pathway [18] , [19] , [20] . PTEN is a non-redundant, plasma membrane lipid phosphatase that antagonizes the PI3K function [21] . Membrane association of PTEN is important, as it dephosphorylates the target phospholipid on the plasma membrane to function [22] , [23] . Ecscr is a transmembrane protein that locates at the plasma membrane and binds to PTEN at its intracellular domain [24] . Hence, Ecscr enhances membrane localization of PTEN, leading to the negative regulation of PI3K/Akt signalling in ECs. In accordance with the crucial role of endothelial PI3K/Akt signalling in angiogenesis, loss of Ecscr substantially enhanced the ischaemia-induced neovascularization [24] . Here we report an unexpected function of Ecscr in the regulation of insulin sensitivity and progression of obesity. We made the serendipitous observation that Ecscr was highly expressed in WAT and BAT, which urged us to investigate its role in the metabolic regulation. Genetic deletion of Ecscr improved glucose tolerance and enhanced insulin sensitivity without changes in body weight (BW) and body fat mass, even under normal chow diet, by modulating insulin signalling in ECs. Moreover, loss of Ecscr led to the concurrent resistance to diet-induced obesity and its related metabolic disorders by enhancing the adipose tissue angiogenesis. Thus, Ecscr may have therapeutic potential for the control of type-2 diabetes and obesity-related metabolic disorders. Ecscr regulates glucose homeostasis and insulin sensitivity We and others previously showed that Ecscr is highly preferentially expressed in ECs [19] , [20] , [25] . During a detailed analysis of Ecscr functions, we found that Ecscr is expressed in adipose tissues at a high level relative to other tissues ( Fig. 1a ). Moreover, Ecscr expression was significantly increased in WAT of obese mice fed a high-fat diet (HFD) compared with that in lean mice ( Supplementary Fig. S1 ). In accordance with the high expression in ECs, Ecscr was largely present in the stromal vascular cells of WAT ( Fig. 1b ). As Ecscr regulates postnatal angiogenesis, this indicates a potential role of Ecscr in adipose tissue angiogenesis. Adipose tissue angiogenesis is an emerging factor in metabolic disorders, and thus we studied mice with a homozygous deletion of Ecscr (Ecscr −/− mice) [24] with respect to glucose homeostasis and energy metabolism. BW, visceral or subcutaneous fat weight, as well as food intake, were similar between Ecscr −/− and wild-type (WT) mice ( Fig. 1c and Supplementary Fig. S2a,b ). No significant difference in BW was also confirmed under a pair-fed condition ( Supplementary Fig. S2c ). We found that blood vessel density in WAT was modestly increased in Ecscr −/− mice relative to WT mice, whereas the vessel density per adipocyte was not different between these mice ( Fig. 1d ). Blood vessel density in BAT was similar between WT and Ecscr −/− mice ( Fig. 1e ). 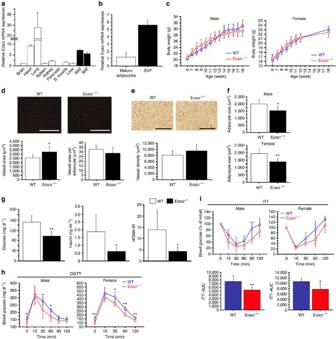Figure 1: Ecscr is expressed in adipose tissues and regulates systemic insulin sensitivity. (a) Expression of Ecscr mRNA relative to 18S levels in mouse tissues fed a normal chow diet (n=3 each). S. muscle, skeletal muscle. (b) Ecscr mRNA expression levels in mature adipocytes and stromal vascular fraction (SVF) of WAT (n=8 each). (c) BW of WT or Ecscr−/−mice at the indicated age (n=8 each for male mice;n=15 each for female mice). (d) Blood vessel density in WAT of WT or Ecscr−/−mice at the age of 20 weeks (n=10 each). Scale bars, 200 μm. (e) Blood vessel density in BAT of WT or Ecscr−/−mice at the age of 20 weeks (n=10 each). Scale bars, 100 μm. (f) Adipocyte size of visceral WAT in WT or Ecscr−/−mice at the age of 20 weeks (n=5 each for male mice;n=8 each for female mice). (g) Fasting blood glucose, serum insulin levels and HOMA-IR in WT and Ecscr−/−mice at the age of 20 weeks (n=6 each). (h,i) OGTT (h) and ITT (i) in WT and Ecscr−/−mice at the age of 20 weeks (n=12 each for male mice;n=6 each for female mice). Area under curve for ITT was also shown (i). *P<0.05, **P<0.01 and ***P<0.001 compared with WT (Student’st-test). All data are mean±s.d. Figure 1: Ecscr is expressed in adipose tissues and regulates systemic insulin sensitivity. ( a ) Expression of Ecscr mRNA relative to 18S levels in mouse tissues fed a normal chow diet ( n =3 each). S. muscle, skeletal muscle. ( b ) Ecscr mRNA expression levels in mature adipocytes and stromal vascular fraction (SVF) of WAT ( n =8 each). ( c ) BW of WT or Ecscr −/− mice at the indicated age ( n =8 each for male mice; n =15 each for female mice). ( d ) Blood vessel density in WAT of WT or Ecscr −/− mice at the age of 20 weeks ( n =10 each). Scale bars, 200 μm. ( e ) Blood vessel density in BAT of WT or Ecscr −/− mice at the age of 20 weeks ( n =10 each). Scale bars, 100 μm. ( f ) Adipocyte size of visceral WAT in WT or Ecscr −/− mice at the age of 20 weeks ( n =5 each for male mice; n =8 each for female mice). ( g ) Fasting blood glucose, serum insulin levels and HOMA-IR in WT and Ecscr −/− mice at the age of 20 weeks ( n =6 each). ( h , i ) OGTT ( h ) and ITT ( i ) in WT and Ecscr −/− mice at the age of 20 weeks ( n =12 each for male mice; n =6 each for female mice). Area under curve for ITT was also shown ( i ). * P <0.05, ** P <0.01 and *** P <0.001 compared with WT (Student’s t -test). All data are mean±s.d. Full size image Interestingly, Ecscr −/− mice showed a small but significant reduction in the size of visceral white adipocytes ( Fig. 1f ). Adipocytes expressed Ecscr at minimal levels in comparison with ECs (Supplementary Fig. S3a), and Ecscr expression was not induced but rather decreased during the adipocyte differentiation of 3T3-L1 pre-adipocytes (Supplementary Fig. S3b). Moreover, loss of Ecscr did not affect the adipogenesis of mouse embryonic fibroblast ( Supplementary Fig. S3c ). These collectively indicate that Ecscr might affect the size of adipocyte in a non-cell autonomous fashion. Despite the comparable BW and body fat mass, Ecscr −/− mice showed reduced fasting blood glucose levels accompanied by lower serum insulin concentration relative to WT mice, resulting in the lower homeostasis model assessment-insulin resistance (HOMA-IR) ( Fig. 1g ). These strongly suggest that Ecscr −/− mice have enhanced insulin sensitivity and, thus, we conducted oral glucose tolerance test (OGTT) and insulin tolerance test (ITT). Elevation of blood glucose after oral glucose administration was significantly reduced and the glucose-lowering effect of insulin was significantly enhanced in Ecscr −/− mice in comparison with that in WT mice, indicating that the inactivation of Ecscr leads to the improved glucose tolerance and enhanced insulin sensitivity even under a normal chow diet ( Fig. 1h,i ). Ecscr modifies the skeletal muscle insulin sensitivity The skeletal muscle blood flow is one of the major determinants in the insulin-mediated glucose uptake and, thus, it regulates the systemic insulin sensitivity [26] , [27] , [28] . Recently, insulin signalling and insulin-mediated eNOS activation in ECs have been shown to have a crucial role in the skeletal muscle insulin sensitivity by regulating the muscle blood flow and insulin delivery into the interstitium of the skeletal muscle [10] . Ecscr modifies the endothelial PI3K/Akt/eNOS signalling [19] , [24] and, therefore, we investigated a role of Ecscr in the insulin-mediated Akt and eNOS activation in ECs. Disruption of Ecscr enhanced the Akt/eNOS signalling without affecting ERK signals in ECs in response to insulin ( Fig. 2a ). Furthermore, insulin-mediated muscle blood flow was significantly enhanced ( Fig. 2b , and Supplementary Movies 1 and 2 ) and the insulin content in the skeletal muscle was increased in Ecscr −/− mice in comparison with those in WT mice ( Fig. 2c ). Consistently, insulin-mediated activation of both insulin receptor (IR)-β and Akt was enhanced in the skeletal muscle of Ecscr −/− mice in comparison with that in WT mice ( Fig. 2d ). Of note, Ecscr expression in the skeletal muscle was relatively low ( Fig. 1a ) and the membrane association of PTEN, which is modified by Ecscr, was similar between WT and Ecscr −/− mice in the skeletal muscle ( Supplementary Fig. S4a ). Moreover, insulin-mediated Akt activation in isolated skeletal muscle was not different between these mice, indicating that insulin signalling in the skeletal muscle was not altered in a cell autonomous fashion by Ecscr deletion ( Supplementary Fig. S4b ). Moreover, the membrane association of PTEN in the liver, insulin signalling in isolated hepatocytes and hepatic gluconeogenetic gene expressions were not different between WT and Ecscr −/− mice ( Supplementary Fig. S4c–e ). 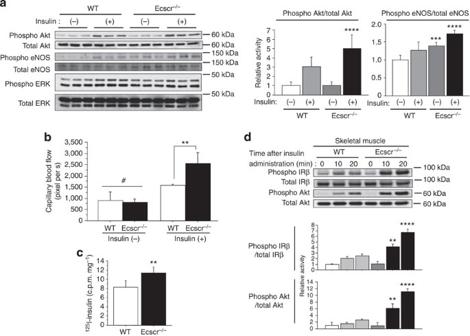Figure 2: Ecscr modifies the endothelial insulin signalling and skeletal muscle insulin sensitivity. (a) Immunoblotting for insulin signals. Aortic EC cells were isolated from WT or Ecscr−/−mice. Cells were stimulated with 1 × 10−7M insulin for 10 min (n=6 each). Full-length images of immunoblots are shown inSupplementary Fig. S15a. (b) Muscle capillary blood flow in WT or Ecscr−/−mice before and after insulin injection (n=5 each). (c) Insulin content in skeletal muscle of WT or Ecscr−/−mice injected with125I-insulin (n=7 each). (d) Activation of insulin receptor-β (IR-β) and Akt was analysed in skeletal muscle of WT or Ecscr−/−mice at indicated times after insulin administration (n=6 each). Full-length images of immunoblots are shown in theSupplementary Fig. S15b.#Not significant, **P<0.01, ***P<0.001 and ****P<0.0001 compared with WT (Student’st-test). All data are mean±s.d. Figure 2: Ecscr modifies the endothelial insulin signalling and skeletal muscle insulin sensitivity. ( a ) Immunoblotting for insulin signals. Aortic EC cells were isolated from WT or Ecscr −/− mice. Cells were stimulated with 1 × 10 −7 M insulin for 10 min ( n =6 each). Full-length images of immunoblots are shown in Supplementary Fig. S15a . ( b ) Muscle capillary blood flow in WT or Ecscr −/− mice before and after insulin injection ( n =5 each). ( c ) Insulin content in skeletal muscle of WT or Ecscr −/− mice injected with 125 I-insulin ( n =7 each). ( d ) Activation of insulin receptor-β (IR-β) and Akt was analysed in skeletal muscle of WT or Ecscr −/− mice at indicated times after insulin administration ( n =6 each). Full-length images of immunoblots are shown in the Supplementary Fig. S15b . # Not significant, ** P <0.01, *** P <0.001 and **** P <0.0001 compared with WT (Student’s t -test). All data are mean±s.d. Full size image We found that the inhibition of NOS by L-NAME abolished the enhanced activation of both IR-β and Akt in response to insulin in the skeletal muscle ( Fig. 3a ). Treatment with L-NAME also abolished the improved glucose tolerance and enhanced systemic insulin sensitivity in Ecscr −/− mice ( Fig. 3b ). Moreover, genetic deletion of eNOS abrogated the increase in insulin-mediated muscle blood flow and also abolished the improved insulin sensitivity observed in Ecscr −/− mice ( Fig. 3c,d ). These collectively indicate that loss of Ecscr improves systemic insulin sensitivity largely through an enhanced skeletal muscle insulin sensitivity by increasing the insulin-mediated eNOS activation in ECs. 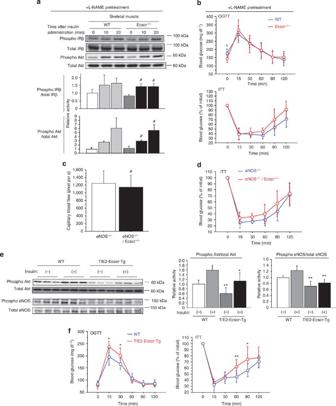Figure 3: Ecscr modifies the insulin sensitivity through a control of insulin-mediated eNOS activation in EC. (a) Immunoblotting for insulin signals. Insulin signalling in skeletal muscle of WT or Ecscr−/−mice pretreated with L-NAME (n=6 each). Full-length images of immunoblots are shown in theSupplementary Fig. S15c. (b) OGTT and ITT in WT or Ecscr−/−mice pretreated with L-NAME (n=8 each). (c) Muscle capillary blood flow in eNOS−/−or eNOS−/−/ Ecscr−/−mice after insulin injection (n=6 each). (d) ITT in eNOS−/−or eNOS−/−/Ecscr−/−mice (n=5 each). (e) Immunoblotting for insulin signals. Aortic ECs from WT or TIE2-Ecscr-Tg (line-1) mice were stimulated with 1 × 10−7M insulin (n=6 each). (f) OGTT and ITT in WT or TIE2-Ecscr-Tg mice (n=8 each).#Not significant compared with WT, *P<0.05 and **P<0.01 compared with WT or eNOS−/−(Student’st-test). All data are mean±s.d. Figure 3: Ecscr modifies the insulin sensitivity through a control of insulin-mediated eNOS activation in EC. ( a ) Immunoblotting for insulin signals. Insulin signalling in skeletal muscle of WT or Ecscr −/− mice pretreated with L-NAME ( n =6 each). Full-length images of immunoblots are shown in the Supplementary Fig. S15c . ( b ) OGTT and ITT in WT or Ecscr −/− mice pretreated with L-NAME ( n =8 each). ( c ) Muscle capillary blood flow in eNOS −/− or eNOS −/− / Ecscr −/− mice after insulin injection ( n =6 each). ( d ) ITT in eNOS −/− or eNOS −/− /Ecscr −/− mice ( n =5 each). ( e ) Immunoblotting for insulin signals. Aortic ECs from WT or TIE2-Ecscr-Tg (line-1) mice were stimulated with 1 × 10 −7 M insulin ( n =6 each). ( f ) OGTT and ITT in WT or TIE2-Ecscr-Tg mice ( n =8 each). # Not significant compared with WT, * P <0.05 and ** P <0.01 compared with WT or eNOS −/− (Student’s t -test). All data are mean±s.d. Full size image To further investigate a role of Ecscr in insulin signalling in ECs, we generated mice in which Ecscr was activated in ECs under the control of Tie2 promoter (TIE2-Ecscr-Tg). As opposed to Ecscr deletion, the targeted activation of Ecscr impeded insulin-mediated Akt and eNOS activation in ECs ( Fig. 3e and Supplementary Fig. S5 ). Notably, TIE2-Ecscr-Tg mice showed modest but significant impairment in glucose tolerance and insulin sensitivity even under a normal chow diet in contrast to Ecscr −/− mice, further supporting a crucial role of endothelial Ecscr in glucose homeostasis ( Fig. 3f ). Genetic deletion of Ecscr protects mice from obesity As adipose tissue angiogenesis has a significant role in the pathogenesis of obesity and its related metabolic disorders, we investigated the role of Ecscr in the progression of obesity. When challenged with an HFD, weight gain was significantly attenuated in Ecscr −/− mice despite the indistinguishable food intake from WT mice ( Fig. 4a,b ). This reduced weight gain in Ecscr −/− mice fed an HFD was also observed even under a pair-fed condition ( Supplementary Fig. S6a ). Visceral and subcutaneous fat weight was lower, and the body fat ratio was significantly reduced in Ecscr −/− mice fed an HFD ( Fig. 4c,d and Supplementary Fig. S6b ). Moreover, hepatic steatosis was ameliorated in Ecscr −/− mice relative to WT mice after an HFD ( Fig. 4e,f ). Furthermore, leptin expression was substantially reduced, whereas adiponectin expression was enhanced in WAT of Ecscr −/− mice fed an HFD ( Supplementary Fig. S7 ). Serum cholesterol level in Ecscr −/− mice was significantly lower than that in WT mice after an HFD, whereas there was no difference in serum cholesterol and triglyceride levels between these mice fed a normal chow diet ( Supplementary Table S1 ). 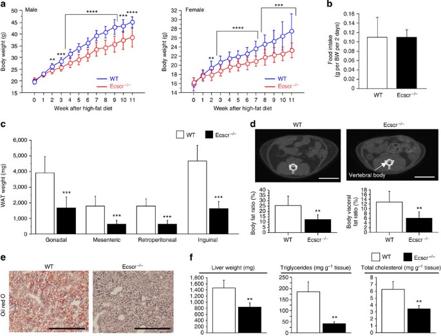Figure 4: Inactivation of Ecscr counteracts diet-induced obesity. (a) BW of WT or Ecscr−/−mice fed an HFD starting at the age of 6 weeks (n=13 for male WT;n=10 for male Ecscr−/−;n=22 for female WT;n=14 for female Ecscr−/−mice). (b) Food intake in WT or Ecscr−/−mice fed an HFD for 12 weeks (n=6 each). (c) Weight of visceral or subcutaneous fat in WT or Ecscr−/−mice fed an HFD for 14 weeks (n=9 each). (d) Body fat ratio assessed by micro CT in WT or Ecscr−/−mice fed an HFD for 12 weeks (n=6 each). Scale bars, 10 mm. (e) Histology of liver stained with Oil Red O in WT or Ecscr−/−mice fed an HFD for 12 weeks. Scale bars, 50 μm. (f) Liver weight and triglycerides or total cholesterol contents in liver of WT or Ecscr−/−mice fed an HFD for 14 weeks (n=5 each). **P<0.01, ***P<0.001 and ****P<0.0001 compared with WT (Student’st-test). All data are mean±s.d. Figure 4: Inactivation of Ecscr counteracts diet-induced obesity. ( a ) BW of WT or Ecscr −/− mice fed an HFD starting at the age of 6 weeks ( n =13 for male WT; n =10 for male Ecscr −/− ; n =22 for female WT; n =14 for female Ecscr −/− mice). ( b ) Food intake in WT or Ecscr −/− mice fed an HFD for 12 weeks ( n =6 each). ( c ) Weight of visceral or subcutaneous fat in WT or Ecscr −/− mice fed an HFD for 14 weeks ( n =9 each). ( d ) Body fat ratio assessed by micro CT in WT or Ecscr −/− mice fed an HFD for 12 weeks ( n =6 each). Scale bars, 10 mm. ( e ) Histology of liver stained with Oil Red O in WT or Ecscr −/− mice fed an HFD for 12 weeks. Scale bars, 50 μm. ( f ) Liver weight and triglycerides or total cholesterol contents in liver of WT or Ecscr −/− mice fed an HFD for 14 weeks ( n =5 each). ** P <0.01, *** P <0.001 and **** P <0.0001 compared with WT (Student’s t -test). All data are mean±s.d. Full size image We then investigated the blood vessel density in WAT and found that vascularization was significantly increased in WAT of Ecscr −/− mice relative to WT mice fed an HFD ( Fig. 5a and Supplementary Fig. S8a ). Moreover, Hypoxyprobe staining revealed a substantially reduced hypoxia in WAT of Ecscr −/− mice fed an HFD ( Fig. 5b ). Of note, macrophage infiltration and expression of inflammatory cytokines in WAT was reduced in HFD-fed Ecscr −/− mice ( Fig. 5c and Supplementary Fig. S8b,c ). As a result, improved glucose tolerance and enhanced insulin sensitivity in Ecscr −/− mice were more evident after an HFD as shown by OGTT and ITT ( Fig. 5d ). These indicate that Ecscr inactivation ameliorates the obesity-related metabolic disorders at least in part by enhancing the adipose tissue angiogenesis in WAT. 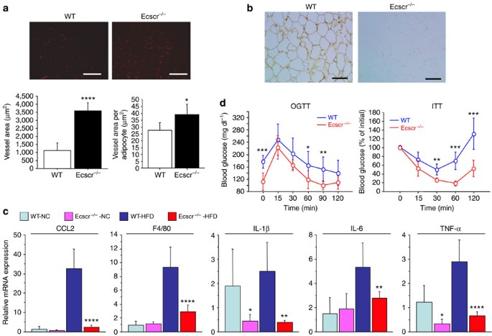Figure 5: Genetic deletion of Ecscr enhances angiogenesis and reduces hypoxia in WAT during an HFD. (a) Blood vessel density in WAT of WT or Ecscr−/−mice fed an HFD for 14 weeks (n=10 each). Scale bars, 100 μm. (b) The presence of hypoxia was investigated by Hypoxyprobe staining in WAT of WT or Ecscr−/−mice fed an HFD for 14 weeks. Hypoxic areas are stained brown. Scale bars, 100 μm. (c) Expression of inflammatory cytokines in WAT of WT or Ecscr−/−mice fed either an normal chow diet (NC) or HFD for 14 weeks (n=8 each). (d) OGTT and ITT were performed in WT or Ecscr−/−mice fed an HFD for 14 weeks (n=7 each). *P<0.05, **P<0.01, ***P<0.001 and ****P<0.0001 compared with WT (Student’st-test). All data are mean±s.d. Figure 5: Genetic deletion of Ecscr enhances angiogenesis and reduces hypoxia in WAT during an HFD. ( a ) Blood vessel density in WAT of WT or Ecscr −/− mice fed an HFD for 14 weeks ( n =10 each). Scale bars, 100 μm. ( b ) The presence of hypoxia was investigated by Hypoxyprobe staining in WAT of WT or Ecscr −/− mice fed an HFD for 14 weeks. Hypoxic areas are stained brown. Scale bars, 100 μm. ( c ) Expression of inflammatory cytokines in WAT of WT or Ecscr −/− mice fed either an normal chow diet (NC) or HFD for 14 weeks ( n =8 each). ( d ) OGTT and ITT were performed in WT or Ecscr −/− mice fed an HFD for 14 weeks ( n =7 each). * P <0.05, ** P <0.01, *** P <0.001 and **** P <0.0001 compared with WT (Student’s t -test). All data are mean±s.d. Full size image In addition, we analysed the expressional changes of various angiogenic factors in adipose tissues in response to the HFD feeding. Expression of angiogenic factors, including vascular endothelial growth factor, was significantly increased in WAT and BAT as early as 2 weeks after an HFD ( Supplementary Fig. S9a ). Of note, the expression of these angiogenic factors did not change in the liver and skeletal muscle even after an HFD ( Supplementary Fig. S9b ). These indicate that HFD feeding initiates the blood vessel remodelling, particularly in adipose tissues. Consistently, blood vessel density in the skeletal muscle and heart was not different between WT and Ecscr −/− mice fed an HFD, in contrast to the increased vascularization in WAT of Ecscr −/− mice ( Supplementary Fig. S10 ). Ecscr deletion enhances thermogenesis and metabolic rate We then investigated the metabolic parameters in HFD-fed WT and Ecscr −/− mice. The oxygen consumption and CO 2 production were greater, whereas the respiratory exchange ratio was reduced in Ecscr −/− mice compared with those in WT mice fed an HFD ( Fig. 6a,b ). In contrast, there was no difference in activity between these mice ( Supplementary Fig. S11 ). These indicate that increased energy expenditure with augmented fat utilization as a source of energy contributes to the resistance to obesity in Ecscr −/− mice. Of note, the core temperature was significantly higher in Ecscr −/− mice than that in WT mice after an HFD ( Fig. 6c ). BAT is a thermogenic organ that makes a major contribution to the overall energy balance [14] , and we found that BAT in HFD-fed Ecscr −/− mice remained in a polygonal shape with eosinophilic in the cytoplasm, whereas that in HFD-fed WT mice lost the typical morphology with large lipid droplets accumulated in the cytoplasm ( Fig. 6d ). Expressions of uncoupling proteins, peroxisome proliferator-activated receptors and genes involved in fatty acid oxidation in BAT of Ecscr −/− mice was enhanced comparing with those in WT mice fed an HFD ( Fig. 6e and Supplementary Fig. S12a ). Moreover, thermogenesis in response to acute cold exposure was substantially augmented in Ecscr −/− mice fed an HFD ( Fig. 6f ). Consistent with the enhanced thermogenesis, fatty acid uptake was considerably increased in BAT of Ecscr −/− mice fed an HFD, whereas the glucose uptake was not altered ( Supplementary Fig. S12b ). As the high thermogenic activity of BAT requires a particularly high rate of blood perfusion, we investigated the blood vessel density in BAT. Vascularization was substantially enhanced and hypoxia was significantly attenuated in BAT of Ecscr −/− mice relative to WT mice after an HFD ( Fig. 6g,h and Supplementary Fig. S13 ). These collectively indicate that Ecscr inactivation enhances thermogenesis by increasing the blood perfusion and oxygen supply in BAT during an HFD, and thus it counteracts the diet-induced obesity. 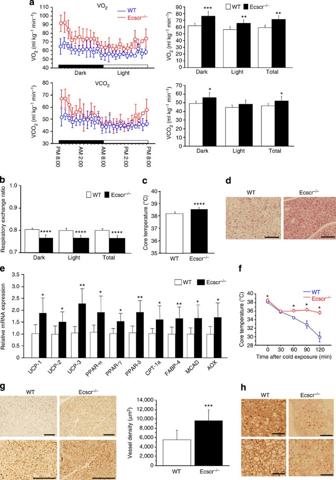Figure 6: Inactivation of Ecscr enhances angiogenesis in BAT and increases thermogenic capacity during an HFD. (a) Oxygen consumption and CO2production in WT or Ecscr−/−mice fed an HFD for 12 weeks (n=6 each). (b) Respiratory exchange ratio in WT or Ecscr−/−mice fed an HFD for 12 weeks. (n=6 each). (c) Core temperature in WT or Ecscr−/−mice fed an HFD for 8 weeks (n=7 for WT;n=10 for Ecscr−/−). (d) Histology of BAT stained with haematoxylin and eosin in WT or Ecscr−/−mice fed an HFD for 14 weeks. Scale bars, 100 μm. (e) Gene expressions in BAT of WT or Ecscr−/−mice fed an HFD for 8 weeks (n=7 each). (f) Core temperature in WT or Ecscr−/−mice fed an HFD for 8 weeks at indicated times after acute cold exposure (n=7 for WT;n=10 for Ecscr−/−). (g) Blood vessel density in BAT of WT or Ecscr−/−mice fed an HFD for 14 weeks (n=10 each). Scale bars, 100 μm. (h) The presence of hypoxia was investigated by Hypoxyprobe staining in BAT of WT or Ecscr−/−mice fed an HFD for 14 weeks. Pictures of two independent WT or Ecscr−/−mice were shown. Hypoxic areas are stained brown. Scale bars, 50 μm. *P<0.05, **P<0.01, ***P<0.001 and ****P<0.0001 compared with WT (Student’st-test). All data are mean±s.d. Figure 6: Inactivation of Ecscr enhances angiogenesis in BAT and increases thermogenic capacity during an HFD. ( a ) Oxygen consumption and CO 2 production in WT or Ecscr −/− mice fed an HFD for 12 weeks ( n =6 each). ( b ) Respiratory exchange ratio in WT or Ecscr −/− mice fed an HFD for 12 weeks. ( n =6 each). ( c ) Core temperature in WT or Ecscr −/− mice fed an HFD for 8 weeks ( n =7 for WT; n =10 for Ecscr −/− ). ( d ) Histology of BAT stained with haematoxylin and eosin in WT or Ecscr −/− mice fed an HFD for 14 weeks. Scale bars, 100 μm. ( e ) Gene expressions in BAT of WT or Ecscr −/− mice fed an HFD for 8 weeks ( n =7 each). ( f ) Core temperature in WT or Ecscr −/− mice fed an HFD for 8 weeks at indicated times after acute cold exposure ( n =7 for WT; n =10 for Ecscr −/− ). ( g ) Blood vessel density in BAT of WT or Ecscr −/− mice fed an HFD for 14 weeks ( n =10 each). Scale bars, 100 μm. ( h ) The presence of hypoxia was investigated by Hypoxyprobe staining in BAT of WT or Ecscr −/− mice fed an HFD for 14 weeks. Pictures of two independent WT or Ecscr −/− mice were shown. Hypoxic areas are stained brown. Scale bars, 50 μm. * P <0.05, ** P <0.01, *** P <0.001 and **** P <0.0001 compared with WT (Student’s t -test). All data are mean±s.d. Full size image Ecscr activation in ECs predisposes mice to obesity To confirm the crucial role of endothelial Ecscr in the Ecscr-mediated metabolic control, we investigated whether the activation of Ecscr in ECs affects the progression of obesity. BW was similar between WT and TIE2-Ecscr-Tg mice fed a normal chow diet ( Supplementary Fig. S14 ). In contrast to Ecscr −/− mice, TIE2-Ecscr-Tg mice were predisposed to diet-induced obesity and they developed aggravated glucose intolerance and insulin resistance compared with WT mice after an HFD ( Fig. 7a–d ). Moreover, the expression of inflammatory cytokines in WAT was enhanced in association with the reduced blood vessel density in HFD-fed TIE2-Ecscr-Tg mice ( Fig. 7e,f ). In addition, leptin expression was increased, whereas adiponectin expression was reduced in WAT of TIE2-Ecscr-Tg mice fed an HFD ( Fig. 7g ). On the other hand, lipid accumulation was aggravated, and expressions of uncoupling proteins, peroxisome proliferator-activated receptors and genes involved in fatty acid oxidation were reduced in BAT of TIE2-Ecscr-Tg mice in comparison with those in WT mice fed an HFD ( Fig. 7h,i ). Core temperature was not significantly different between HFD-fed WT and TIE2-Ecscr-Tg mice under ambient condition, but thermogenesis in response to acute cold exposure was impaired in HFD-fed TIE2-Ecscr-Tg mice ( Fig. 7j ). Moreover, TIE2-Ecscr-Tg mice fed an HFD showed the reduced vascularization in BAT ( Fig. 7k ). These indicate that targeted activation of Ecscr in ECs aggravated diet-induced obesity and its related metabolic disorders by reducing the adipose tissue angiogenesis in WAT and BAT. 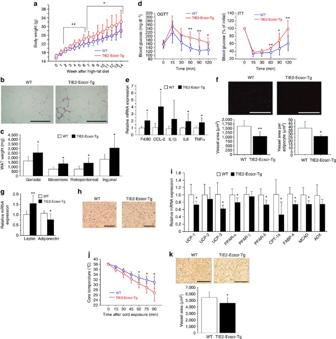Figure 7: Targeted activation of Ecscr in EC predisposes mice to obesity. (a) BW of WT or TIE2-Ecscr-Tg female mice fed an HFD starting at the age of 6 weeks (n=10 for WT;n=12 for Tg mice). (b) Histology of WAT stained with haematoxylin and eosin in WT or TIE2-Ecscr-Tg mice fed an HFD for 14 weeks. Scale bars, 200 μm. (c) Visceral or subcutaneous fat weight in WT or TIE2-Ecscr-Tg mice fed an HFD for 14 weeks (n=7 each). (d) OGTT and ITT in WT or TIE2-Ecscr-Tg mice fed an HFD for 14 weeks (n=7 each). (e) Expression of inflammatory cytokines in WAT of WT or TIE2-Ecscr-Tg mice fed an HFD for 14 weeks (n=7 each). (f) Blood vessel density in WAT of WT or TIE2-Ecscr-Tg mice fed an HFD for 14 weeks (n=10 each). Scale bars, 200 μm. (g) The expression of leptin and adiponectin in WAT of WT or TIE2-Ecscr-Tg mice fed an HFD for 14 weeks (n=7 each). (h) Histology of BAT stained with haematoxylin and eosin in WT or Ecscr−/−mice fed an HFD for 14 weeks. Scale bars, 100 μm. (i) Gene expressions in BAT of WT or TIE2-Ecscr-Tg mice fed an HFD for 14 weeks (n=7 each). (j) Core temperature in WT or TIE2-Ecscr-Tg mice fed an HFD for 12 weeks at indicated times after acute cold exposure (n=6 each). (k) Blood vessel density in BAT of WT or TIE2-Ecscr-Tg mice fed an HFD for 14 weeks (n=10 each). Scale bars, 100 μm. *P<0.05 and **P<0.01 compared with WT (Student’st-test). All data are mean±s.d. Figure 7: Targeted activation of Ecscr in EC predisposes mice to obesity. ( a ) BW of WT or TIE2-Ecscr-Tg female mice fed an HFD starting at the age of 6 weeks ( n =10 for WT; n =12 for Tg mice). ( b ) Histology of WAT stained with haematoxylin and eosin in WT or TIE2-Ecscr-Tg mice fed an HFD for 14 weeks. Scale bars, 200 μm. ( c ) Visceral or subcutaneous fat weight in WT or TIE2-Ecscr-Tg mice fed an HFD for 14 weeks ( n =7 each). ( d ) OGTT and ITT in WT or TIE2-Ecscr-Tg mice fed an HFD for 14 weeks ( n =7 each). ( e ) Expression of inflammatory cytokines in WAT of WT or TIE2-Ecscr-Tg mice fed an HFD for 14 weeks ( n =7 each). ( f ) Blood vessel density in WAT of WT or TIE2-Ecscr-Tg mice fed an HFD for 14 weeks ( n =10 each). Scale bars, 200 μm. ( g ) The expression of leptin and adiponectin in WAT of WT or TIE2-Ecscr-Tg mice fed an HFD for 14 weeks ( n =7 each). ( h ) Histology of BAT stained with haematoxylin and eosin in WT or Ecscr −/− mice fed an HFD for 14 weeks. Scale bars, 100 μm. ( i ) Gene expressions in BAT of WT or TIE2-Ecscr-Tg mice fed an HFD for 14 weeks ( n =7 each). ( j ) Core temperature in WT or TIE2-Ecscr-Tg mice fed an HFD for 12 weeks at indicated times after acute cold exposure ( n =6 each). ( k ) Blood vessel density in BAT of WT or TIE2-Ecscr-Tg mice fed an HFD for 14 weeks ( n =10 each). Scale bars, 100 μm. * P <0.05 and ** P <0.01 compared with WT (Student’s t -test). All data are mean±s.d. Full size image Ecscr rescue in ECs reverses the metabolic phenotypes To further confirm that EC is the primary target in Ecscr-mediated metabolic control, we performed rescue-type experiments by crossing the TIE2-Ecscr-Tg and Ecscr −/− mice. Endothelial-specific re-expression of Ecscr completely abolished the enhanced insulin sensitivity in Ecscr −/− mice fed a normal chow diet ( Fig. 8a ). Moreover, re-expression of Ecscr in ECs reversed the ameliorated diet-induced obesity and abrogated the enhanced adipose tissue angiogenesis observed in Ecscr −/− mice fed an HFD ( Fig. 8b–d ). 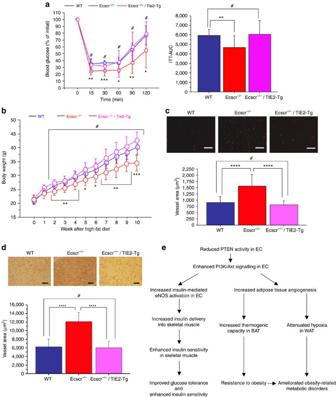Figure 8: Endothelial re-expression of Ecscr reverses metabolic phenotypes of Ecscr−/−mice. (a) ITT and area under curve for ITT in WT, Ecscr−/−or Ecscr−/−/TIE2-Tg mice fed an NC (n=7 each). (b) BW of WT, Ecscr−/−or Ecscr−/−/TIE2-Tg mice fed an HFD starting at the age of 6 weeks (n=8 each). (c) Blood vessel density in WAT of WT, Ecscr−/−or Ecscr−/−/TIE2-Tg mice fed an HFD for 10 weeks (n=10 each). Scale bars, 100 μm. (d) Blood vessel density in BAT of WT, Ecscr−/−or Ecscr−/−/TIE2-Tg mice fed an HFD for 10 weeks (n=10 each). Scale bars, 100 μm. (e) Proposed mechanisms for the enhanced insulin sensitivity and resistance to obesity induced by Ecscr inactivation. Inactivation of Ecscr enhances systemic insulin sensitivity through the augmented insulin-mediated PI3K/Akt/eNOS signalling in EC. Moreover, the loss of Ecscr protects mice from obesity and its related metabolic disorders through the enhanced adipose tissue angiogenesis during an HFD due to the augmented PI3K/Akt signalling in EC.#Not significant, *P<0.05, **P<0.01, ***P<0.001 and ****P<0.0001 compared with WT (one-way analysis of variance). All data are mean±s.d. Figure 8: Endothelial re-expression of Ecscr reverses metabolic phenotypes of Ecscr −/− mice. ( a ) ITT and area under curve for ITT in WT, Ecscr −/− or Ecscr −/− /TIE2-Tg mice fed an NC ( n =7 each). ( b ) BW of WT, Ecscr −/− or Ecscr −/− /TIE2-Tg mice fed an HFD starting at the age of 6 weeks ( n =8 each). ( c ) Blood vessel density in WAT of WT, Ecscr −/− or Ecscr −/− /TIE2-Tg mice fed an HFD for 10 weeks ( n =10 each). Scale bars, 100 μm. ( d ) Blood vessel density in BAT of WT, Ecscr −/− or Ecscr −/− /TIE2-Tg mice fed an HFD for 10 weeks ( n =10 each). Scale bars, 100 μm. ( e ) Proposed mechanisms for the enhanced insulin sensitivity and resistance to obesity induced by Ecscr inactivation. Inactivation of Ecscr enhances systemic insulin sensitivity through the augmented insulin-mediated PI3K/Akt/eNOS signalling in EC. Moreover, the loss of Ecscr protects mice from obesity and its related metabolic disorders through the enhanced adipose tissue angiogenesis during an HFD due to the augmented PI3K/Akt signalling in EC. # Not significant, * P <0.05, ** P <0.01, *** P <0.001 and **** P <0.0001 compared with WT (one-way analysis of variance). All data are mean±s.d. Full size image Taken together, Ecscr modifies the systemic insulin sensitivity, the progression of obesity and its related metabolic disorders largely through a modification of EC functions ( Fig. 8e ). In the present study, we demonstrated that Ecscr provides a previously undescribed mode of regulation in energy metabolism and glucose homeostasis. Genetic loss of Ecscr enhanced the systemic insulin sensitivity and concurrently counteracts diet-induced obesity. Until recently, there have been only a few reports of genetically modified mice that show enhanced insulin sensitivity under normal diet and concomitant resistance to diet-induced obesity [29] , [30] . The striking difference of Ecscr −/− mice from these mice is that the enhanced insulin sensitivity under normal diet arises in the absence of leanness in Ecscr −/− mice. This unique metabolic phenotype of Ecscr −/− mice is due to the roles of Ecscr in both endothelial insulin signalling and adipose tissue angiogenesis. PTEN/PI3K pathway has a central role in insulin signalling and, therefore, this pathway has been an attractive pharmacotherapeutic target to modulate insulin sensitivity to treat type-2 diabetes. Nevertheless, systemic regulation of this pathway is not feasible, because it evokes crucial and universal cellular functions in a variety type of cells. Genetic loss of PTEN or catalytic subunit of PI3K causes fetal death in utero , indicating their essential roles during the embryonic development [31] , [32] , [33] . Moreover, systemic reduction in PTEN levels induces cancer susceptibility [31] , [34] . Ecscr modifies PTEN function by regulating its membrane association and it shows highly preferential expression in ECs. Hence, the regulation of Ecscr could provide a partial and cell type-specific modification of PTEN function. Therefore, the inhibition of Ecscr offers a unique therapeutic potential without inducing detrimental conditions, such as oncogenicity, yet it still possibly accelerates the growth of pre-existent tumours through enhanced angiogenesis. Ecscr −/− mice fed a normal chow showed modest reduction in adipocyte size, but its underlying mechanisms remain to be elucidated. The expression of Ecscr in adipocytes was minimal, and Ecscr expression was not induced but rather decreased during the adipocyte differentiation in 3T3-L1 pre-adipocytes. Furthermore, loss of Ecscr did not affect the adipocyte differentiation, indicating that Ecscr does not directly regulate the adipogenesis in a cell autonomous fashion. On the other hand, it has been reported that ECs and/or angiogenesis enhances pre-adipocyte proliferation and differentiation into mature adipocyte, and thus promotes adipogenesis [35] , [36] . As the blood vessel density in WAT was increased in Ecscr −/− mice, we presume that the smaller size of adipocyte observed in Ecscr −/− mice might be associated with the increased blood vessel density in WAT. Ecscr −/− mice were resistant to diet-induced obesity due to the increased energy expenditure with augmented utilization of fat as a source of energy. Higher core temperature concomitant with the enhanced thermogenic capacity strongly suggests that increased energy expenditure is due to the enhanced thermogenesis. Enhanced palmitate uptake, as well as increased expression of uncoupling proteins, peroxisome proliferator-activated receptors and genes involved in fatty acid oxidation in BAT, further corroborates the enhanced thermogenesis in HFD-fed Ecscr −/− mice. These findings were associated with the enhanced vascularization and reduced hypoxia in BAT, and therefore the increased angiogenic function in ECs of BAT largely contributes to the resistance to obesity in Ecscr −/− mice, although a molecular link between angiogenesis and the mitochondrial gene expression in BAT is still unclear. Further experiments using UCP1-deficient mice would be helpful to strengthen the BAT activation in HFD-fed Ecscr −/− mice. Moreover, increased vascularization and reduced hypoxia in WAT contributes to the ameliorated obesity-related metabolic disorders at least in part in HFD-fed Ecscr −/− mice by reducing the adipose tissue inflammation. As previous data showed the highly preferential expression of Ecscr in ECs [19] , [20] , [25] , we presume that Ecscr expression in most tissues reflects its expression in ECs. Reverse effects of the targeted Ecscr activation in ECs on systemic insulin sensitivity and progression of obesity, especially in mice with Ecscr-null background, strongly suggest that Ecscr regulates glucose homeostasis and energy metabolism largely by modulating EC functions. Nevertheless, we cannot exclude the possibility of a minor expression of Ecscr in insulin target cells other than ECs, and without the EC-specific gene deletion study the possibility that part of the metabolic effects observed in Ecscr −/− mice are due to altered signalling in other cell types still remains. Experiments using mice with EC-specific Ecscr deletion in the future would certainly strengthen our conclusion. Endothelial insulin signalling controls insulin delivery particularly in the skeletal muscle, because of the continuous capillary structure of the muscle [37] , [38] , [39] . Accordingly, enhanced insulin-mediated eNOS activation in the EC led to the increased muscle capillary blood flow and enhanced the insulin delivery into the skeletal muscle in Ecscr −/− mice. On the other hand, under an HFD, enhanced angiogenesis in WAT and BAT of Ecscr −/− mice also contributes to the reduced insulin resistance by attenuating the hypoxia-mediated chronic inflammation in WAT, as well as by increasing the thermogenesis in BAT. Notably, enhanced angiogenesis in response to the HFD feeding was initiated specifically in adipose tissues but not the other tissues examined. These collectively make the effects of Ecscr deletion selective to adipose tissues and skeletal muscle, and thus enhanced PI3K/Akt/eNOS signalling in ECs is the primary mechanism for the improved insulin sensitivity in Ecscr −/− mice fed both a normal chow and an HFD. Our data established Ecscr as a new factor in the pathogenesis for insulin resistance and obesity, and shed light on the EC-mediated regulation in the systemic energy metabolism and glucose homeostasis. Enhancing the insulin sensitivity without increasing BW is a major challenge for the treatment of type-2 diabetes. Recent studies with positron emission tomography/computed tomography (CT) scanning using 18 F-fluorodeoxyglucose have shown the presence of metabolically active BAT that contributes to energy expenditure in adult human [40] . Therefore, the inhibition of Ecscr potentially improves insulin sensitivity and concurrently counteracts obesity in human as well, and thus Ecscr represents an attractive target for the control of metabolic disorders, although its role in other PTEN-controlled biological processes remains to be elucidated. Materials Phospho-Akt (Ser473), Akt, phospho-eNOS (Ser1177), phospho-p44/42 MAPK (ERK1/2), ERK1/2, phospho-IR-β (Tyr1146), IR-β, PTEN antibodies were purchased from Cell Signaling Technology. Antibody for eNOS was purchased from Santa Cruz Biotechnology. Glyceraldehyde 3-phosphate dehydrogenase antibody was purchased from Upstate Biotechnology. F4/80 antibody was purchased from Abcam. Cell culture 3T3-L1 pre-adipocytes were obtained from the Health Science Research Resources Bank (Japan). Adipogenesis was induced as described previously [41] . Briefly, confluent 3T3-L1 pre-adipocytes were treated with insulin, dexamethasone and isobutylmethylxanthine at day 0 for 48 h, followed by the treatment with insulin for another 48 h. Afterwards, cells were cultured in the growth medium (DMEM supplemented with 10% fetal bovine serum). ECs were isolated from mouse aorta and were cultured as reported previously [42] . Briefly, the aorta from adult C57BL/6 mice were cut into 1-mm-thick rings and placed in 24-well culture plates, and were cultured in EGM2-MV medium (Clonetics). ECs that sprouted out of the aortic rings were passaged for one to two times before use for experiments. Aortic ECs were cultured in the medium supplemented with 1% fetal bovine serum for 12 h before the stimulation with insulin. Hepatocytes were isolated and cultured as reported previously [43] . Briefly, mouse liver was perfused with perfusion medium containing collagenase (type-I), followed by plating on culture plates coated with collagen-I. Cells were starved by culturing in serum-free medium for 12 h before the stimulation with insulin. Animal study All experimental protocols were approved by the Ethics Review Committee for Animal Experimentation of Kyoto Prefectural University of Medicine. Targeting of the Ecscr gene in mice was performed as reported previously [24] . In the knockout allele, exon 1–3 of Ecscr were replaced with the Neo cassette. Transgenic mice were generated, which overexpressed Ecscr in ECs under the control of the Tie2 promoter (TIE2-Ecscr-Tg). The plasmid containing the Tie2 promoter and enhancer was a kind gift from Thomas N Sato (Nara Institute of Science and Technology, Japan). The TIE2-Ecscr-Tg mice were propagated as heterozygous Tg animals by bleeding with WT C57BL6/J mice. Male and female mice were fed either a normal chow diet (containing 23.1% protein and 5.1% fat) or a HFD (Oriental Bio HFD-60 that contains 35% fat, 25.3% carbohydrate and 23% protein). For the HFD feeding, mice at the age of 6 weeks were maintained on an HFD for up to 14 weeks. For the pair-feeding study, Ecscr −/− mice at the age of 6 weeks were allowed feed ad libitum , and the control WT mice at the same age were pair-fed the same amount of food as was consumed by the Ecscr −/− mice. Isolation of mature adipocytes from WAT Adipocytes and non-adipocytes were prepared by the collagenase method from epididymal adipose tissue of 20-week-old mice on a normal chow diet as reported previously [44] . Briefly, the tissue homogenates were fractionated by brief centrifugation (350 g for 20 s) in Krebs–Henseleit 4-(2-hydroxyethyl)-2-piperazine ethanesulphonic acid buffer (pH 7.4) supplemented with 20 mg ml −1 of BSA (fraction V) and 2 mmol l −1 of glucose. Floating cells were mature adipocytes, and pelleted cells were used as stromal vascular fraction. Insulin signalling studies In female mice, 0.75 U kg −1 insulin or saline was injected subcutaneously. The soleus muscle was removed at the indicated times and was immediately lysed in RIPA buffer. In some experiments, mice were treated with 3 mM L-NAME (Sigma) in drinking water for 1 week before the experiments. Metabolic measurements Food intake and oxygen consumption (VO 2 ) was determined in 18-week-old mice fed an HFD for 12 weeks with an O 2 /CO 2 metabolic measuring system (Muromachi CO., Ltd, Japan) as reported previously [45] , [46] . VO 2 was determined when the minimum plateau shape was obtained during the light cycle, which corresponded to the period of sleep or inactivity. VO 2 is expressed as the volume of O 2 consumed per kilogram weight per minute. Rectal temperature was monitored with an electronic thermometer (Model BAT 12R, Bio Research Center, Japan) equipped with a rectal probe (Model RET-3). For the acute cold exposure experiments, 14-week-old mice fed an HFD for 8 weeks were housed single mouse per cage and were kept at 4 °C. The rectal temperature was measured at indicated times after acute cold exposure. The OGTT and ITT were performed as reported previously [45] , [46] . Briefly, for the OGTT, mice were fasted for 6 h and D -glucose at 2 g kg −1 (mice fed a normal chow diet) or 0.5 g kg −1 (mice fed an HFD) was orally administered. For the ITT, mice were given human insulin at 0.75 U kg −1 (mice fed a normal chow diet) or 1 U kg −1 (mice fed an HFD) by subcutaneous injection. Blood glucose was measured by the glucose oxidase method (Sanwa Kagaku, Japan). Serum insulin concentration was measured by ELISA assay. Histological analysis Target tissues were extracted following perfusion fixation with 4% paraformaldehyde. Specimens were further fixed with 4% paraformaldehyde and then embedded with paraffin. Adipose tissue sections were stained with haematoxylin and eosin, with anti-F4/80 antibody to detect macrophage, or with isolectin GS-IB4 from Griffonia Simplicifolia (Invitrogen) to detect capillaries as reported previously [47] . Briefly, sections were incubated with anti-F4/80 antibody (1:100 dilution) or isolectin-IB4 (1:200 dilution) at 4 °C overnight, following blocking with PBS containing 5% normal goat serum for 1 h. F4/80-positive or isolectin-positive cells were quantified at two randomly chosen independent fields/each section. Liver tissues were embedded in OCT compound (Sakura Finetech, Japan) and were snap-frozen followed by staining sections with Oil Red O. Quantification of blood vessel density and immunostainings Blood vessel density and immunostain-positive areas were measured by using the NIH image software as previously reported [48] , [49] . Briefly, images of stained sections were extracted by colour-split function of the software. Thereafter, the stain-positive area was measured automatically by the NIH image. Analysis with Hypoxyprobe Adipose tissue hypoxia was analysed according to a standard protocol using Hypoxyprobe-1 kit (Hypoxyprobe, Inc.) as reported previously [16] . Briefly, the Hypoxyprobe was administered by intraperitoneal injection. After 1 h, adipose tissues were excised and fixed with 4% paraformaldehyde, followed by embedding with paraffin. Hypoxia was detected by immunohistochemistry analysis using anti-Hypoxyprobe antibody. Immunoblotting Cell lysates were prepared in RIPA buffer, and then immunoblotting was performed as described previously [50] . Briefly, lysates containing the same amount of proteins underwent SDS–PAGE, followed by transferring onto the nitrocellulose membrane. Membranes were incubated with specific antibody to detect target molecules. Detailed information for antibodies is described in Supplementary Table S2 . In some experiments, membranes were cut into two to three pieces, to detect several target molecules in one blot without the stripping process (for example, the IR, Akt and glyceraldehyde 3-phosphate dehydrogenase). When the phosphorylation of target molecules was analysed, total and phosphorylated forms were detected using the same membrane, but in some experiments different blots prepared in the same way at the same time were used because of the low affinity of the antibodies. Preparation of membrane fraction Isolated liver or skeletal muscle specimens were put in ice-cold homogenization buffer containing 250 mM sucrose, 20 mM phosphate buffer (pH6.8), protease inhibitor cocktail (Sigma) and phosphatase inhibitors. Skeletal muscle specimens were treated with collagenase to remove connective tissues before the procedure. Tissues were homogenized gently on ice using a Dounce tissue grinder (Sigma) and centrifuged at 1,000 g for 10 min to remove nuclei and remaining cells. The supernatants were ultracentrifuged at 150,000 g for 30 min using an Optima TLX (Beckman) with TLA 100.3 rotor. The supernatants were collected as the cytosol fraction. Pellets were lysed with RIPA buffer and centrifuged, and the supernatants were obtained as the membrane fraction. Quantitative RT–PCR Total RNA was extracted by using Trizol (Invitrogen) followed by purification with RNeasy MiniElute cleanup kit (Invitrogen). Complementary DNA was synthesized from 2 to 5 μg of total RNA using SuperScript first-strand synthesis system (Invitrogen). PCR reactions were prepared by using LightCycler FastStart DNA Masterplus SYBR Green I (Roche Applied Science) followed by the real-time PCR using LightCycler (Roche Applied Science) or by using CYBR Premie Ex TaqII (TaKaRa, Japan) followed by the real-time PCR using Thermal Cycler Dice (TaKaRa). Nucleotide sequence of each primer is shown in Supplementary Tables S3 and S4 . Target genes mRNA levels relative to β-actin was shown unless otherwise described. CT scan analysis The body fat ratio was investigated radiographically using CT (LaTheta, ALOKA) according to the manufacturer’s protocol. CT scanning was performed at 2-mm intervals from the diaphragm to the bottom of the abdominal cavity. Measurement of the skeletal muscle capillary blood flow The skeletal muscle capillary blood flow was measured as reported previously [10] , with a minor modification. The hindlimb muscles were imaged in the short axis using a 30-MHz transducer (RMV 704) connected to an ultrasound system (Vevo 2100; VisualSonics Inc.). Sonazoid (Daiichi Sankyo Corporation), which consists of an aqueous dispersion of lipid-stabilized perfluorobutane-filled gas microbubbles, was infused before or 10 min after insulin administration. Then, images were immediately collected for 10 s to assess the enhancement. The capillary blood volume filled with microbubbles was measured by using ImageJ software. Briefly, moving images were imported as 228 frames of still pictures, and each picture was subtracted with the mean intensity image calculated by the software. The remaining images represent the microbubble contrast agent and the area of which was measured for each picture frames. Measurement of insulin content in skeletal muscle Mice were injected with 0.75 U kg −1 insulin that contains 125 nCi ml −1 I 125 -labelled insulin (PerkinElmer). After 5 min, circulating blood was washed out with 10 ml PBS, and soleus muscle was extracted. The radioactivity of the extracted muscle was measured by using γ-counter. Measurement of glucose and palmitate uptake The amount of radio-labelled glucose and palmitate to administer to mice was determined according to the previous report [51] , [52] . Mice fed an HFD were intravenously injected with 800 nCi 14 C-glucose and 20 nCi 3 H-palmitate. After 10 min, circulating blood was washed out with 10 ml PBS, and then the heart, liver, WAT, BAT and soleus muscle were extracted. The radioactivity of the extracted organs was measured by using scintillation counter. Statistical analysis All data are presented as mean±s.d. Differences between groups were analysed by Student’s t -test or one-way analysis of variance with post hoc multiple comparison by Bonferroni/Dunn test. P <0.05 was considered statistically significant. How to cite this article: Akakabe, Y. et al . Ecscr regulates insulin sensitivity and predisposition to obesity by modulating endothelial cell functions. Nat. Commun. 4:2389 doi: 10.1038/ncomms3389 (2013).